Non-volatile optoelectronic memory based on a photosensitive dielectric Recently, the optoelectronic memory is capturing growing attention due to its integrated function of sense and memory as well as multilevel storage ability. Although tens of states have been reported in literature, there are still three obvious deficiencies in most of the optoelectronic memories: large programming voltage (>20 V), high optical power density (>1 mW cm −2 ), and poor compatibility originating from the over-reliance on channel materials. Here, we firstly propose an optoelectronic memory based on a new photosensitive dielectric (PSD) architecture. Data writing and erasing are realized by using an optical pulse to switch on the PSD. The unique design enables the memory to work with a programming voltage and optical power density as low as 4 V and 160 µW cm −2 , respectively. Meanwhile, this device may be extended to different kinds of transistors for specific applications. Our discovery offers a brand-new direction for non-volatile optoelectronic memories with low energy consumption. The emergence of smart home, autonomous driving, and bionic robots etc. marks the arrival of big data era, which puts forward increasingly higher requirements for nonvolatile memory, one of the carriers of information storage [1] . Flash memory has always been in an unshakable position in nonvolatile memory field [2] , [3] , [4] , although some new structures or principles, such as magnetic random-access memory [5] , ferroelectric random-access memory [6] , phase-change memory [7] and resistive random-access memory [8] , were constantly proposed. However, faced with the already-arrived big data era, the drawbacks of flash memory have gradually emerged. Firstly, general flash memory cell has a two-state storage capacity, and the integration density is being restricted by the scaling down limit [9] , which creates a huge gap between the considerable data generated every day and the existing storage capability. Secondly, the programming voltage of flash memory has been maintained above 10 V, leading to a huge energy consumption [4] . The reason lies in its core structure and programming process, as shown in Fig. 1a, b . The difference between the flash memory and the common metal–oxide–semiconductor field-effect transistor (MOSFET) is the insertion of a 9–10 nm tunneling dielectric (TD) layer and a floating gate (FG) surrounded by the dielectric layers. Writing or erasing data depends on the electrons’ transport through the TD layer back and forth via Fowler–Northeim tunneling [10] process and the resulting shift of the threshold voltage, which inevitably requires a large gate voltage ( V GS ) pulse (Fig. 1b ). Fig. 1: Difference between flash memory and PSD-based optoelectronic memory in terms of the device structure and write and erase processes. a Flash memory structure. b Write and erase processes in the flash memory. c Structure of the PSD-based optoelectronic memory. d Write and erase processes in the PSD-based optoelectronic memory. The solid balls represent the electrons, and the hollow balls represent the holes. The arrows represent flow directions of electrons or holes. Full size image The property of electrical read-out orthogonal to the photo-programming operation promises high differentiation among different data levels and imparts the ability of multilevel storage to optoelectronic memory [9] . For instance, different electrical signals, namely multi-states, can be obtained by adjusting the wavelength, the pulse width, the pulse number, the optical power density and even the polarization of the optical pulse. Currently, three storage mechanisms were mainly adopted in optoelectronic memories: photochromic effect [10] , defects trapping of photogenerated carriers [11] , [12] , [13] , [14] , [15] , [16] , [17] , and tunneling of photogenerated carriers [1] , [18] , [19] . For photochromic memories, high optical power density is essential to break or connect the bonds in the polymer materials and modulate their resistance. A high-programming voltage is then a major requisite for the electrical regulation of the polymers. In the case of defects trapping in channel or interface, the photogenerated carriers will be captured in the defects and released slowly after turning off the optical pulse, known as persistent photoconductivity (PPC) effect. Because only a fraction of photogenerated carriers can be trapped by defects, the high optical intensity is needed to provide enough photogenerated carriers. Meanwhile, a large V GS needs to be exerted to release the carriers trapped by the defects. The third-type memory device utilizes the tunneling of the photogenerated carriers in channel through the TD to FG under the large V GS . Similarly, because the probability of tunneling is small, the high optical power density is needed to provide enough photogenerated carriers into the channel. As discussed above, a situation of high energy consumption will be inevitably encountered, considering the fact that the programming voltage and optical power density used in the previously reported optoelectronic memories were in excess of 20 V and 1 mW m −2 , respectively. In addition, the strong dependence of these structures on the selection of channel materials and the control of defects makes it difficult to adapt to certain situations with different channel materials. It is urgently needed to develop new storage structure and working principle to realize the optoelectronic memory with low energy consumption and improved compatibility. Design of novel optoelectronic memory based on the PSD A new optoelectronic memory structure with a photosensitive dielectric (PSD) is designed on the basis of the flash memory cell. As shown in Fig. 1c , the original normal dielectric (ND) layer in the flash memory (Fig. 1a ) is replaced with a PSD layer, and the TD layer between the FG and the channel is replaced with an ND layer. Critically, the dielectric layer instead of the channel serves as the photosensitive component. The new PSD should own three significant features—(i) it works as a dielectric layer in dark, that is, it is insulating; (ii) it acts as a semiconductor and produce photogenerated carriers under illumination; (iii) it forms a distinct band offset with the FG layer and offers an energy barrier sufficient to block the carriers trapped in the FG. It can be recognized that, with the assistance of an optical excitation with a suitable wavelength matching the bandgap of the PSD layer, the injection of electrons will be achieved by applying a small negative V GS pulse, as indicated by the green arrows in Fig. 1d . Under the illumination, the photogenerated electrons in the PSD layer will drift to the FG layer driven by the negative V GS . After turning off the optical pulse, the PSD immediately becomes insulating, and the electrons in the FG are bound in the potential well formed by the energy barriers between the PSD, FG, and ND separately. In this case, the threshold voltage ( V th ) of the transistor will positively shift [2] , therefore accomplishing the writing and storage process of “0” state. Correspondingly, extraction of electrons will be achieved by applying a small positive V GS pulse combined with a similar optical pulse, as indicated by the red arrows in Fig. 1d . The electrons bounded in the FG will easily transport across the original barrier between the FG and PSD due to illumination-induced conductivity change in the PSD layer. Once stopping the optical pulse, the PSD immediately becomes insulating again, no electrons stay in the FG, and the threshold voltage will shift to the negative direction, erasing the “0” state and storaging “1” state. In contrast to the optoelectronic memory reported in literature, the PSD-based memory introduces an innovative approach of injecting and extracting carriers with low power consumption as well as avoiding tradeoffs with choosing specific channel materials. The first and foremost, since the programming voltage is only used to guide the transport direction of the photogenerated carriers originated from the PSD, its value does not need to be large. Another outstanding merit of the new architecture is the efficient use of the intrinsic excitation-generated carriers in PSD for charge storage. It will remarkably decrease the need for a high optical power density. Thirdly, photogenerated carriers are generated in the PSD layer rather than in the general channel layer. It indicates that this new idea may feasibly work in different types of transistors, with less selectivity for channel materials (e.g., Si, oxides, 2D materials). The fabrication and performance of the novel PSD-based optoelectronic memory The key for realizing the designed structure and mechanism is to find a suitable PSD material that exhibits the above-mentioned three features. Recently, Ga 2 O 3 ultra-wide bandgap semiconductor ( ∼ 5.0 eV [20] ) has attracted considerable attention in the solar-blind UV detection research field [20] , [21] , [22] , [23] . Zheng et al. [24] and Kaya et al. [25] reported the use of Ga 2 O 3 a the high-K dielectric layer for MOSFETs in 2007 and 2016, respectively. It should be noticed that the electron affinity of Ga 2 O 3 is ~4 eV, which enables the formation of a sufficiently high band offset between Ga 2 O 3 and metals with high work function, such as Au having the work function of 5.2 eV [26] . These data suggest that Ga 2 O 3 may satisfy all tradeoffs as the PSD we are looking for. To start with, we prepared a two-terminal vertical structure based on Ga 2 O 3 , which is the top and core part of the PSD-based optoelectronic memory. The schematic diagram and top view of the magnified micrograph of the fabricated device are shown in Fig. 2a and Supplementary Fig. S1 , respectively. Note that no diffraction peaks were observed in the XRD curve of the Ga 2 O 3 film (Supplementary Fig. S2 ), proving the amorphous nature of the Ga 2 O 3 deposited by radio-frequency magnetron sputtering at room temperature. Figure 2b demonstrates the core level spectra of O 1 s and Ga 3 d measured by X-ray photoelectron spectroscopy (XPS), and Ga:O atomic ratio approaches 2:3 determined by the ratio of the integrated photoelectron peak area of O 1 s to Ga 3 d . 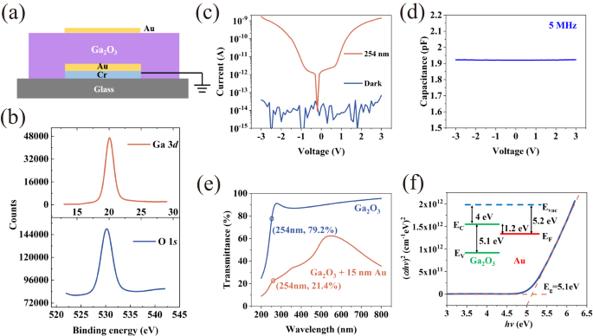Fig. 2: Characterization of the vertical structure based on Ga2O3film. aSchematic diagram of the vertical structure.bXPS spectra of the Ga2O3film. The upper and lower panels show the core level spectra of Ga 3dand O 1s.cI–V curves in dark (blue curve) and under 254 nm illumination (orange curve).dC–V sweep curve at 5 MHz.eOptical transmittance spectra of the Ga2O3(45 nm) film (blue curve) and the Ga2O3(45 nm) + Au (15 nm) film (orange curve).fThe plot of (αhν)2versushν for Ga2O3film. The inset is the energy band structure of Ga2O3and Au. It suggests fewer oxygen vacancy defects in the Ga 2 O 3 film and thus lower dark current in the device [23] . As shown in Fig. 2c , the dark current of the vertical structure is maintained at the ∼ 10 −14 A level, which is basically the limit of the source meter. In addition, a C–V test is conducted on the vertical structure at 5 MHz (Fig. 2d ) and a relative permittivity value is extracted as 13.01, which shows that Ga 2 O 3 can work as an insulating dielectric layer. The transmission spectrum of the Ga 2 O 3 film is illustrated in Fig. 2e , with a direct bandgap of ~5.1 eV by Tauc’s law, as shown in Fig. 2f . It means that the Ga 2 O 3 film has strong absorption for light whose wavelength locates at around 250 nm. Correspondingly, an apparent photoresponse is observed in Ga 2 O 3 under 254 nm irradiation (Fig. 2c ), satisfying the second requirement of the PSD as a semiconductor under suitable illumination. In addition, to decrease the absorption of control gate (CG) in the final device (Fig. 1c ), 15 nm half-transparent Au was deposited on Ga 2 O 3 as CG. The result manifests that about 50% of light is still absorbed and reflected by the top CG (Fig. 2e ). Fig. 2: Characterization of the vertical structure based on Ga 2 O 3 film. a Schematic diagram of the vertical structure. b XPS spectra of the Ga 2 O 3 film. The upper and lower panels show the core level spectra of Ga 3 d and O 1 s . c I–V curves in dark (blue curve) and under 254 nm illumination (orange curve). d C–V sweep curve at 5 MHz. e Optical transmittance spectra of the Ga 2 O 3 (45 nm) film (blue curve) and the Ga 2 O 3 (45 nm) + Au (15 nm) film (orange curve). f The plot of (α h ν) 2 versus h ν for Ga 2 O 3 film. The inset is the energy band structure of Ga 2 O 3 and Au. Full size image For the ultimate demonstration, we constructed a top-gate InGaZnO (IGZO) thin film transistor (TFT), the bottom part of the PSD-based optoelectronic memory. The schematic diagram and the top view magnified micrograph of the fabricated device are shown in Supplementary Fig. S3a, S3b , respectively. The initial linear region of the output characteristic curve (Supplementary Fig. S3c ) clearly indicates the formation of a good ohmic contact between the source/drain electrodes and the channel. The transfer characteristic curve (Supplementary Fig. S3d ) shows that the device has normal TFT performance with a high on-off ratio (>10 8 ), which is the precondition for a large memory window. The two-terminal Ga 2 O 3 vertical structure and top-gate IGZO TFT are stacked together to compose the final PSD-based optoelectronic memory device. Figure 3a, b show the schematic diagram and top view of the magnified micrograph of the final device, respectively. 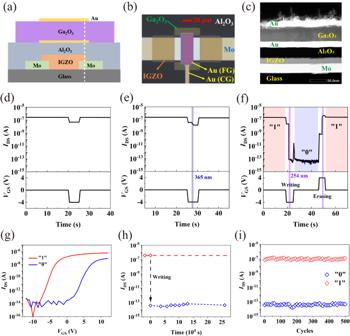Fig. 3: The structure and performance of the final PSD-based optoelectronic memory device. aSchematic diagram of the device.bTop view of the magnified optical micrograph of the fabricated device.cTEM cross-sectional image corresponding to the position of the white dashed line in (a).dThe writing result byVGS= −4 V pulse.eThe writing result by a combination ofVGS= −4 V pulse and a 365 nm of 160 µW cm−2optical pulse.fThe single write/erase process and corresponding results. (optical pulse: 254 nm, 160 µW cm−2, 1 s;VGSpulse: −4V / 4 V).gTransfer characteristic curves in states “0” and “1”.hRetention test for up to 72 h. (optical pulse: 254 nm, 160 µW cm−2, 1 s;VGSpulse: −4 V).iFatigue test result for 500 cycles. (optical pulse: 254 nm, 160 µW cm−2, 1 s;VGSpulse: −4 V/4 V).g–iBlue represents “0”, and red represents “1”. Figure 3c is the cross-sectional TEM image, where Au, Ga 2 O 3 , Au, Al 2 O 3 , IGZO, and Mo layers are clearly observed exhibiting sharp interfaces. To avoid the possible contaminations of the photoresist at the interfaces, each lithography process is optimized as shown in Supplementary Fig. S4 . Importantly, the band alignment of this memory structure matches the new conception introduced in Fig. 1d , as confirmed in Supplementary Fig. S5 . Fig. 3: The structure and performance of the final PSD-based optoelectronic memory device. a Schematic diagram of the device. b Top view of the magnified optical micrograph of the fabricated device. c TEM cross-sectional image corresponding to the position of the white dashed line in ( a ). d The writing result by V GS = −4 V pulse. e The writing result by a combination of V GS = −4 V pulse and a 365 nm of 160 µW cm −2 optical pulse. f The single write/erase process and corresponding results. (optical pulse: 254 nm, 160 µW cm −2 , 1 s; V GS pulse: −4V / 4 V). g Transfer characteristic curves in states “0” and “1”. h Retention test for up to 72 h. (optical pulse: 254 nm, 160 µW cm −2 , 1 s; V GS pulse: −4 V). i Fatigue test result for 500 cycles. (optical pulse: 254 nm, 160 µW cm −2 , 1 s; V GS pulse: −4 V/4 V). g – i Blue represents “0”, and red represents “1”. Full size image The transfer characteristics of the PSD-based optoelectronic memory (Supplementary Fig. S6 ) basically retain the performance of the isolated IGZO TFT, except slightly larger subthreshold swing ( SS ) value and more negative threshold voltage ( V th ). That is ascribed to a smaller capacitance caused by the series connection of the two capacitors (CG/PSD/FG + FG/ND/channel) in the device. It is clearly demonstrated that only applying negative V GS pulses is not sufficient to inject charges into the FG, as shown in Fig. 3d , as there is no light to turn on the PSD. Moreover a combination of the negative V GS pulse with a 365 nm optical pulse cannot cause the carriers’ injection either (Fig. 3e ), since 365 nm does not match the bandgap of Ga 2 O 3 . The single writing and erasing process and their results are shown in Fig. 3f to verify the memory function of the final device. V GS and the drain voltage ( V DS ) under read status were 0 V and −0.5 V, respectively. In the initial state “1”, the drain current ( I DS ) is stably maintained at ~3 × 10 −7 A. After applying a V GS pulse = −4 V and a 254 nm optical pulse with as low as 160 µW cm −2 power, I DS is stably maintained at ~5 × 10 −14 A, corresponding to “0” state with a memory window >10 6 . As expected, the electrons are injected into the FG from the CG and trapped in the FG in this process, causing a right shift of the threshold voltage ( Fig. 3g ). Then we apply a V GS = 4 V pulse and an identical optical pulse, and the I DS recovered to the initial value, ~3 × 10 −7 A. The phenomenon indicates that after the 254 nm light “turns on” Ga 2 O 3 , the electrons stored in the FG are rapidly released back to the CG under the electric field induced by the small positive V GS and net electrons in FG. Apparently, the electrons’ transport direction can be discerned from the synchronous variation of the gate current ( I GS ) during the writing and erasing operations of I DS , as shown in Supplementary Fig. S7 . During the writing process, the negative I GS (process “B”) proves that electrons flow from CG to FG, while the positive I GS (process “C”) proves that electrons flow from FG to CG during the erasing process. The in-situ monitoring results of the electrons’ transport behavior perfectly is in accordance with the designed injection/extraction processes highlighted by green and red arrows in Fig. 1d , solidly corroborating the feasibility of the working principle in PSD-based optoelectronic memory. The data retention time is an important parameter of the device reliability. As shown in Fig. 3h , the memory window constantly keeps >10 6 even after 72 h. The original data of retention test are shown in Supplementary Fig. S8 . Fatigue characteristic is another important parameter of the device reliability. The cyclic program/erase (P/E) endurance of the device was examined and exhibited in Fig. 3i . After 500 cycles, the memory window has almost not changed. Compared with conventional three-terminal transistor devices, the addition of optical pulse provides a new route to multilevel storage in nonvolatile memories. Here, three different methods are explored to illustrate the multilevel storage capability. First, we change the amplitude of the V GS pulse to implement multilevel storage. As shown in Fig. 4a , the more negative V GS is, the more electrons are injected into the FG, and the lower I DS is. During the 15 min retention test, every state keeps stable. Figure 4b shows the transfer curves corresponding to every state. 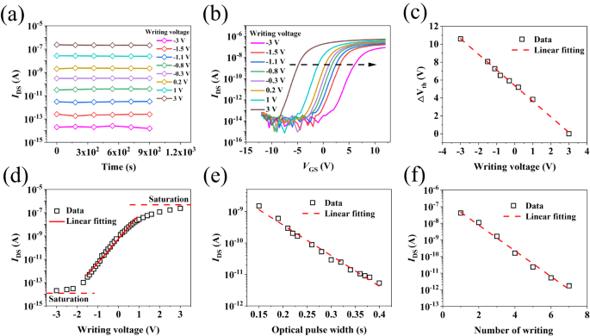Fig. 4: Tests of the multilevel storage. aRetention test of different states formed by differentVGSpulses (keeping the optical pulse at 254 nm, 160 µW cm−2, 1 s). The corresponding relationship between color and writing voltage is shown in the legend.bTransfer curves of different states formed by differentVGSpulses. The corresponding relationship between color and writing voltage is shown in the left legends.cLinear fitting of ∆Vth for different states formed by differentVGSpulse. TheVthis defined as the value ofVGSwhenIDS= (W/L) × 1 nA,WandLare width and length of the channel, respectively.dLinear fitting ofIDSfor different states formed by differentVGSpulse.eLinear fitting ofIDSfor different states formed by different optical pulse width (optical pulse: 254 nm, 160 µW cm−2;VGSpulse: −4 V).fLinear fitting ofIDSfor different states formed by different number of writing (optical pulse: 254 nm, 60 µW cm−2, 50 ms;VGSpulse: −3 V). The more negative the V GS is, the more the curve right shifts. Figure 4c shows that V th shifts (∆ V th ) extracted from Fig. 4b have a good linear relationship with the amplitude of V GS pulse. Linear fitting result of I DS for different states indicates in a write voltage between −2 V and 1 V, corresponding to a current storage window range of approximately 6 orders of magnitude, we can obtain a large number of linearly related storage states, as shown in Fig. 4d . Then, by changing the optical pulse width and the number of writings, we can also obtain a linearly related multilevel storage states, as shown in Fig. 4e , f . Fig. 4: Tests of the multilevel storage. a Retention test of different states formed by different V GS pulses (keeping the optical pulse at 254 nm, 160 µW cm −2 , 1 s). The corresponding relationship between color and writing voltage is shown in the legend. b Transfer curves of different states formed by different V GS pulses. The corresponding relationship between color and writing voltage is shown in the left legends. c Linear fitting of ∆ V th for different states formed by different V GS pulse. The V th is defined as the value of V GS when I DS = ( W / L ) × 1 nA, W and L are width and length of the channel, respectively. 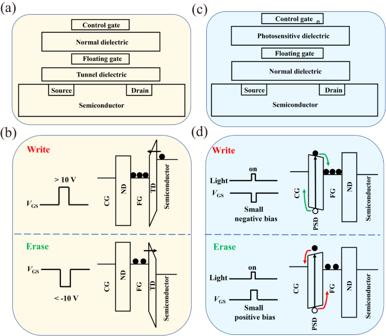d Linear fitting of I DS for different states formed by different V GS pulse. e Linear fitting of I DS for different states formed by different optical pulse width (optical pulse: 254 nm, 160 µW cm −2 ; V GS pulse: −4 V). f Linear fitting of I DS for different states formed by different number of writing (optical pulse: 254 nm, 60 µW cm −2 , 50 ms; V GS pulse: −3 V). Fig. 1: Difference between flash memory and PSD-based optoelectronic memory in terms of the device structure and write and erase processes. aFlash memory structure.bWrite and erase processes in the flash memory.cStructure of the PSD-based optoelectronic memory.dWrite and erase processes in the PSD-based optoelectronic memory. The solid balls represent the electrons, and the hollow balls represent the holes. The arrows represent flow directions of electrons or holes. Full size image Table 1 compares key parameters of the PSD-based optoelectronic memory proposed by us with previously reported ones. The new memory exhibits comparable performance regarding memory window, retention time, and fatigue cycles. The programming voltage and optical power density are particularly far lower than those ever-reported values, which reveals the contribution of PSD in the novel structure. Table 1 Comparison of key parameters with previously reported optoelectronic memories Full size table To get closer to the practical application, we use an AlGaN UV-LED [27] as the light source to realize the programming function of the PSD-based optoelectronic memory. The electroluminescence spectrum of the UV-LED is shown in Supplementary Fig. S9a . The photograph of the test configuration is exhibited in Supplementary Fig. S9b . As seen from these data, the function of writing and erasing has been successfully achieved by using the combination of AlGaN UV-LED and Ga 2 O 3 PSD-based optoelectronic memory (Supplementary Fig. S9c ). This demonstration paves the way for future integration of optoelectronic memory circuits. The optoelectronic memory with IGZO as a channel and Ga 2 O 3 as the PSD is the first example of PSD-based device architecture not only conceptually proposed, but also tested in experimental conditions. It paves the way to explore more PSD candidates and various channel materials. In addition, the memory performance can be further optimized. For instance, longer retention and faster writing speed may be potentially achieved by reducing the defect in PSD. By optimizing the SS parameter of the transistor, a larger memory window can be obtained under the same write conditions, or a smaller programming voltage and optical power density be obtained under the same memory window. The number of multilevel storages can also increase with more subdivided write methods or larger memory windows. In summary, with the booming development of ultra-wide-bandgap semiconductors, the boundary between semiconductors and insulators has become more and more blurred. Here, Ga 2 O 3 is opted as the PSD material in novel nonvolatile optoelectronic memory, considering its admirable insulating property in dark and semiconducting performance under illumination. Via integrating the Ga 2 O 3 PSD with the common floating gate device, unique programming methods are established with low programming voltage (4 V), low optical power density (160 µW cm −2 ), and multilevel storage (storage window of approximately six orders of magnitude with good linear relationship). This memory may potentially fill the gap between big data and limited storage capacity as well as reducing the energy consumption. Meanwhile, the new structure and mechanism can be readily extended to other FETs compatible with photolithography, such as Si-based, organic or 2D materials-based FETs, to achieve high-performance solid-state memory and flexible memory. Remarkably, the device can also be used as a multi-function sensor, integrating the sensing and storage abilities together [28] , [29] . Preparation of a two-terminal vertical structure based on Ga 2 O 3 First, the glass substrate is sonicated with acetone, alcohol, and deionized water for 10 min in sequence. After drying the glass substrate with nitrogen, 10 nm Cr layer is deposited by radio-frequency (RF) magnetron sputtering to improve the adhesion of Au (32 nm) on glass, followed by using photolithography and etching into bottom electrode pattern. Then Ga 2 O 3 (45 nm) is deposited by RF magnetron sputtering (60 W) in an oxygen-rich condition, and 15 nm Au is then sputtered on Ga 2 O 3 . Patterning of the top electrode and gallium oxide is completed in sequence. Finally, the device is annealed at 200 °C for 30 min in air. Preparation of IGZO top-gate TFT First, use the same method to clean the glass substrate. Then grow Mo (30 nm) by magnetron sputtering, and define the channel length (20 µm) and width (50 µm) by photolithography. Then grow IGZO (20 nm) by RF magnetron sputtering. After IGZO is patterned, Al 2 O 3 (30 nm) is grown by atomic layer deposition (ALD) at 200 °C. Then Au (15 nm) is deposited by RF magnetron sputtering. After that, Au is etched to form the gate pattern, and the aluminum oxide is etched to expose the source and drain electrodes for testing. Similarly, the device is annealed at 200 °C for 30 min in air. Preparation of PSD-based optoelectronic memory device Based on the TFT manufacturing process, the original Au (10 nm) is etched to form the FG pattern. Then follow the same method to grow 45 nm Ga 2 O 3 as the PSD layer and 15-nm semitransparent Au as the CG. Finally, Au, Ga 2 O 3 and Al 2 O 3 are etched in sequence. Similarly, the device is annealed at 200 °C for 30 min in air. Material characterization The XPS measurements were conducted using a multifunctional X-ray Photoelectron Spectroscopy analysis platform (ESCALAB Xi + , ThermoFisher), where an electron source was used for charge compensation. TEM cross-sectional image was obtained by TEM (JEM-F200). The transmission spectrum was measured by UV–Vis–NIR Spectrophotometer (UH4150, Hatachi). The XRD curve was measured by an X-ray diffractometer (D8-ADVANCE, Bruker). Device characterization Except for C–V test performed by Keysight B1500A and current source of AlGaN UV-LED provided by Keithley 2400, all other electrical tests were conducted by Keithley 2636B. The light source other than the LED is generated by an UV-enhanced xenon lamp, and the wavelength is adjusted by a monochromator. The generation of optical pulses is achieved by placing an electric switch between the xenon lamp and the monochromator. The optical power density is calibrated by a standard Si photodetector.